Iridium oxide nanotube electrodes for sensitive and prolonged intracellular measurement of action potentials Intracellular recording of action potentials is important to understand electrically-excitable cells. Recently, vertical nanoelectrodes have been developed to achieve highly sensitive, minimally invasive and large-scale intracellular recording. It has been demonstrated that the vertical geometry is crucial for the enhanced signal detection. Here we develop nanoelectrodes of a new geometry, namely nanotubes of iridium oxide. When cardiomyocytes are cultured upon those nanotubes, the cell membrane not only wraps around the vertical tubes but also protrudes deep into the hollow centre. We show that this nanotube geometry enhances cell-electrode coupling and results in larger signals than solid nanoelectrodes. The nanotube electrodes also afford much longer intracellular access and are minimally invasive, making it possible to achieve stable recording up to an hour in a single session and more than 8 days of consecutive daily recording. This study suggests that the nanoelectrode performance can be significantly improved by optimizing the electrode geometry. Two major classes of electrophysiology methods, intracellular and extracellular recording, have been developed to measure action potentials with complementary capabilities. Traditional intracellular recording methods such as whole-cell patch clamp requires rupturing a portion of the plasma membrane to access the cell interior directly [1] . Whole-cell patch clamp is the most sensitive method to record action potentials but is highly invasive and difficult to implement, which precludes long-term or large-scale recording. On the other hand, extracellular recording methods such as multi-electrode arrays utilize micropatterned electrodes to afford noninvasive, long-term and multiplexed measurements [2] , [3] , [4] . For the sake of these gains, however, extracellular recording suffers significantly in signal strength and quality. Therefore it is unsuitable for sensitive measurements such as the shape of the action potential, which contains crucial information about the type, the state and the density of various ion channels [1] . In cardiomyocytes, ion channel dysfunction and deregulation are involved in many cardiac diseases [5] . The shape of the action potential is also an important indicator of the cell type and the maturation stage of the stem cell-derived cardiomyocytes [6] , [7] , [8] . Currently intracellular recording is still the only technique for sensitive measurement such as the duration, the refractory period and the upstroke velocity of the action potentials [7] . This has resulted in the ongoing development of electrophysiological methods with the goal to combine the advantages of both intracellular and extracellular recording methods [9] , [10] , [11] . In the past few years, there have been development of techniques that aim at achieving intracellular recording with extracellular nanoelectrodes or transistors [12] , [13] , [14] , [15] . In particular, extracellular vertical nanoelectrodes have been shown to be able to gain intracellular access upon localized membrane electroporation and able to detect intracellular action potentials with good signal-to-noise ratio [12] , [13] , [16] . These studies identified that the vertical geometry is crucial for the enhanced signal detection because the cell membrane wraps tightly around the vertical electrodes, leading to a reduction of the membrane–electrode gap distance and higher seal resistance [16] , [17] , [18] ( Fig. 1a ). Although intracellular recording by nanopillar electrode possesses unique advantages of minimal invasiveness and easy scalability, it is still limited by signal loss at the membrane–electrode gap. In addition, the time duration of its intracellular access after electroporation is severely limited to just a few minutes because of spontaneous membrane repair [12] , [13] , [15] , [19] . 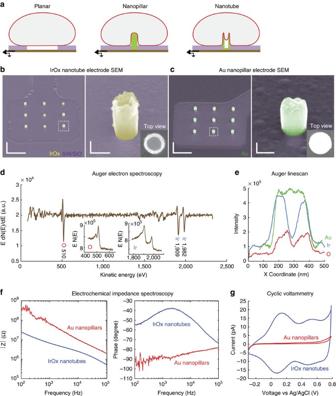Figure 1: Characterization of vertical IrOx nanotube electrode. (a) Schematics of cells interfacing with planar, vertical nanopillar and vertical nanotube electrodes. The cell membrane not only wraps around the outside of the nanotube but also protrudes inside the hollow centre. (b) SEM images of a three-by-three array of IrOx nanotubes on a square Pt pad with the rest of the area insulated with Si3N4/SiO2. The hollow centre of the nanotube can be clearly seen in expanded 52° tilted view and the top view. Scale bars, left 2 μm, right 200 nm. (c) SEM images of Au nanopillar electrodes show solid pillars. The diameter of the Au nanopillar is designed to be slightly larger than the IrOx nanotube so that they have similar surface area. Scale bars, left 2 μm, right 200 nm. (d) Auger electron spectrum of the nanotube electrodes confirms the presence of iridium and oxygen (insets: raw spectra). (e) Elemental line scans along the diameter of an IrOx nanotube and a Au nanopillar. Ir and O plots (blue and red) show two peaks at the sidewall and a drop at the centre, while Au (green) shows a flat top. (f) Electrochemical impedance spectroscopy of IrOx nanotube and Au nanopillar electrodes in phosphate-buffered saline. (g) Cyclic voltammetry of IrOx nanotube and Au nanopillar electrodes in PBS at a scan rate of 30 mV s−1. Figure 1: Characterization of vertical IrOx nanotube electrode. ( a ) Schematics of cells interfacing with planar, vertical nanopillar and vertical nanotube electrodes. The cell membrane not only wraps around the outside of the nanotube but also protrudes inside the hollow centre. ( b ) SEM images of a three-by-three array of IrOx nanotubes on a square Pt pad with the rest of the area insulated with Si 3 N 4 /SiO 2 . The hollow centre of the nanotube can be clearly seen in expanded 52° tilted view and the top view. Scale bars, left 2 μm, right 200 nm. ( c ) SEM images of Au nanopillar electrodes show solid pillars. The diameter of the Au nanopillar is designed to be slightly larger than the IrOx nanotube so that they have similar surface area. Scale bars, left 2 μm, right 200 nm. ( d ) Auger electron spectrum of the nanotube electrodes confirms the presence of iridium and oxygen (insets: raw spectra). ( e ) Elemental line scans along the diameter of an IrOx nanotube and a Au nanopillar. Ir and O plots (blue and red) show two peaks at the sidewall and a drop at the centre, while Au (green) shows a flat top. ( f ) Electrochemical impedance spectroscopy of IrOx nanotube and Au nanopillar electrodes in phosphate-buffered saline. ( g ) Cyclic voltammetry of IrOx nanotube and Au nanopillar electrodes in PBS at a scan rate of 30 mV s −1 . Full size image We seek to further increase the signal amplitude and prolong intracellular access duration by modifying the geometry of the recording nanoelectrodes. We take advantage of previous observations that the cell membrane not only curves inward to wrap around nano-objects but also protrudes outward into nanoholes as small as 100 nm diameter [20] , [21] . In this work, we engineer vertical iridium oxide (IrOx) nanotube electrodes that promote the spontaneous wrapping of the cell membrane around the outside of the nanotube and also its protrusion into the hollow centre ( Fig. 1a ). IrOx is a proven material with high biocompatibility [22] , [23] , [24] , [25] . We show that such strong attachment between the plasma membrane and the IrOx nanotube electrodes leads to an increase in the recorded signal amplitude and one-to-two orders of magnitude increase of the intracellular access duration, compared with Au nanopillar electrodes having the same surface area. Fabrication and characterization of IrOx nanotube electrodes IrOx nanotube electrodes were fabricated in three steps. The first step patterns the underlying Pt lines for electrical connection and insulates them with Si 3 N 4 /SiO 2 . The second step defines the nanotube locations by creating nanoholes using electron beam lithography followed by etching through the Si 3 N 4 /SiO 2 insulation layer. And the third step creates the IrOx nanotubes by electrodeposition of IrOx into pre-defined nanoholes ( Supplementary Fig. 1 ). The small array footprint of 4 × 4 μm 2 allows single cell recording. While electrodeposition of metals gives solid nanopillar geometry, electrodeposition of IrOx yields nanotubes with hollow centres [26] , [27] , [28] . The left images in Fig. 1b,c show a three-by-three array of vertical IrOx nanotube electrodes and Au nanopillars electrodes connected to the underlying Pt pads, respectively. The hollow core of the IrOx nanotubes is obvious from the expanded side and top views ( Fig. 1b , right image), while the Au electrodes appear as solid nanopillars ( Fig. 1c , right image). Supplementary Fig. 2 shows that the nanotubes are uniform with 181±3 nm diameter (peak-to-peak) and 40±3 nm wall thickness ( n =30), and their height is ~500 nm and can be tuned by template thickness and electrodeposition duration. The nanotubes are sealed on their bottom ends by a layer of IrOx contacting the Pt pads ( Supplementary Fig. 3 ). The diameter of the Au nanopillar of ~300 nm is designed to be slightly larger than the IrOx nanotube so that they have the same surface area in contact with the solution (calculated IrOx nanotube surface area of 0.57 μm 2 compared with Au nanopillar surface area of 0.54 μm 2 ). An Auger electron spectrum of the nanotube shows characteristic peaks for oxygen and iridium [29] and thus confirms that the nanotubes are made of IrOx ( Fig. 1d and see Supplementary Fig. 4 for Au nanopillars). Elemental analysis line scans of the nanotubes along their diameter shows two peaks for the sidewall and a drop at the hollow centre (blue and red lines in Fig. 1e ). The spatial overlap of the oxygen and iridium spectra further indicates the uniformity of chemical composition. In comparison, a line scan of a solid Au nanopillar shows a flat top (green line in Fig. 1e ). Electrochemical studies reveal that IrOx nanotube electrodes have lower impedance and a higher charge storage capacity than Au nanopillars of the same surface area. Electrochemical impedance spectroscopy shows that the impedance of IrOx nanotubes (|Z|=5.8±1.1 MΩ at 1 kHz) is an order of magnitude smaller than that of Au nanopillars (|Z|=86.9±22.0 MΩ at 1 kHz) in phosphate-buffered saline ( Fig. 1f ). Phase scan indicates that IrOx nanotubes behave as parallel capacitor-resistor circuits while Au nanopillars with a −90° phase behave similar to perfectly capacitive electrodes ( Fig. 1f ). Cyclic voltammetry ( Fig. 1g ) also shows that the total charge storage capacity of IrOx nanotubes (30.3±1.6 mC cm −2 ) is similar to that of electrodeposited IrOx film [22] , [23] and much larger than the capacity of Au nanopillars (0.69±0.07 mC cm −2 ). The large charge storage capability makes IrOx a superior material for electric stimulation purpose [22] , [28] . For recording purpose, 6 × 6 μm 2 planar IrOx and Au electrodes measure similar extracellular action potentials, even though the IrOx electrode records less noise ( Supplementary Fig. 5 ). Sensitive recording of intracellular action potentials We used IrOx nanotube electrodes for intracellular recording of HL-1 rat cardiomyocytes and primary rat cardiomyocytes. The substrate surface was coated with fibronectin in gelatin solution for cell adhesion [30] and no other surface functionalization was performed to enhance cell membrane adhesion to the electrodes [14] or facilitate electrode penetration into the cell bodies [31] , [32] . Cell survival measurement showed that there is no distinction among cell viability on day 3 and 7 on Au film, Au nanopillar arrays, IrOx film and IrOx nanotube arrays ( Supplementary Fig. 6 ). Rat HL-1 and primary cardiomyocytes were cultured on nanotube electrodes for 3–5 days before electrophysiology measurement (illustrated in Fig. 2a ). Spontaneous and rhythmic mechanical contractions were visible under a bright field microscope and small extracellular action potentials could be detected ( Fig. 2b ). After delivering a train of electric pulses (see Methods section for parameters), the nanotube electrodes gained electrical access to the cell interior by local electroporation. Immediately afterwards, the nanotube electrodes recorded up to 15 mV of rhythmic intracellular action potentials ( Fig. 2c ). The beating interval remained unchanged before and after electroporation (the percentage change is (−0.51±1.45)%, n =22 cells). Measurements over many cells confirmed that nanotube electrodes recorded larger signal than gold nanopillars of similar surface area ( Fig. 2c,d ). For the signal amplitude comparison, we restricted our measurements to cells that had been beating ~3 Hz for at least two days as the recorded amplitude and beating interval vary depending on cell culture age [12] , [30] . The initial action potentials recorded by the IrOx nanotube electrodes ( n =40) were in the range of 1.5–15 mV. At the same conditions, Au nanopillars ( n =33) recorded intracellular action potentials in the range of 0.8–3 mV. Intracellular recording of primary cardiomyocytes shows similar results ( Supplementary Fig. 7 ). 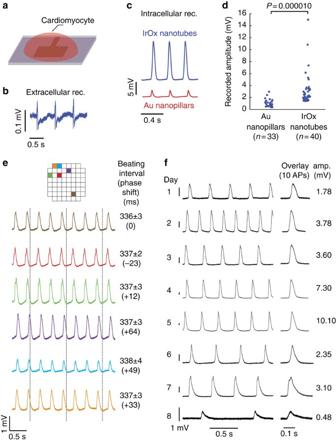Figure 2: Intracellular recording of action potentials by the IrOx nanotube electrodes. (a) Schematic illustration of electrophysiology recording using vertical IrOx nanotube electrodes. (b) Before local electroporation, nanotube electrodes measured extracellular action potentials in HL-1 cardiomyocytes. (c) Immediately after local electroporation, both IrOx nanotube and Au nanopillar achieved intracellular recording of action potentials. (d) Statistical measurements show that nanotube electrodes recorded much larger signal than nanopillars of similar surface area. (e) Simultaneous recording by six different nanotube electrode arrays in the same culture. Adjacent array separation is 100 μm and the array positions on the chip are colour labelled. The vertical dashed lines are guides to see the phase shift of action potentials among different electrodes. (f) Intracellular recording of a single cell over eight consecutive days (the lifespan of the culture). Figure 2: Intracellular recording of action potentials by the IrOx nanotube electrodes. ( a ) Schematic illustration of electrophysiology recording using vertical IrOx nanotube electrodes. ( b ) Before local electroporation, nanotube electrodes measured extracellular action potentials in HL-1 cardiomyocytes. ( c ) Immediately after local electroporation, both IrOx nanotube and Au nanopillar achieved intracellular recording of action potentials. ( d ) Statistical measurements show that nanotube electrodes recorded much larger signal than nanopillars of similar surface area. ( e ) Simultaneous recording by six different nanotube electrode arrays in the same culture. Adjacent array separation is 100 μm and the array positions on the chip are colour labelled. The vertical dashed lines are guides to see the phase shift of action potentials among different electrodes. ( f ) Intracellular recording of a single cell over eight consecutive days (the lifespan of the culture). Full size image IrOx nanotubes are also robust electrodes that offer parallel recording as well as multiple-day monitoring of single cells throughout the lifespan of the cultures. Since the IrOx nanotubes are built upon planar electrode array architecture, they can perform simultaneous recording of multiple cells in a culture. Figure 2e shows a recording by six different electrodes on an 8 × 8 array chip with 100 μm separation between adjacent electrodes. The identical beating interval reveals that the whole culture underwent synchronized beating. Furthermore, our IrOx nanotube electrodes can monitor the action potential evolution in the same cell over eight consecutive days ( Fig. 2f ), which is the lifespan of the culture [30] . The initial increase in recorded action potential amplitude and frequency reflects culture maturation while the subsequent decrease of amplitude and frequency reflects culture ageing. This experiment shows that intracellular recording by nanotube electroporation is minimally invasive. In addition, Supplementary Fig. 8 shows the six-consecutive-day recording by the same electrode in a different culture, demonstrating that the IrOx nanotube electrodes are robust for repeated experiments. Nanotube electrodes drastically increase recording durations Electroporation-induced access to cell interior is transient because of the spontaneous membrane resealing [33] , [34] . Previous measurements using Pt nanopillars [12] and gold mushroom-shaped microelectrodes [19] demonstrated that the cell membrane reseals in just a few minutes after electroporation, which severely limits the time duration of intracellular recording by nanoelectrodes (see Supplementary Note 1 ). In agreement with previous studies, our gold nanopillars electrodes showed that the amplitude of recorded action potentials decayed quickly, often in less than 1 min ( Fig. 3a ). Action potentials recorded by IrOx nanotubes in this period were stable after electroporation and showed no decay. 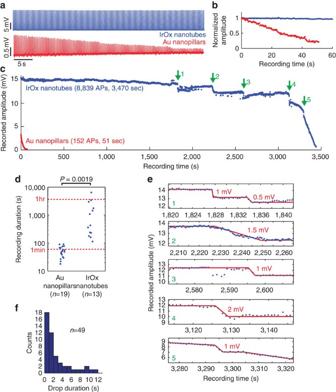Figure 3: Prolonged intracellular access duration by IrOx nanotube electrodes. (a) Intracellular recording of HL-1 action potentials by IrOx nanotube and Au nanopillar electrodes for the first 60 s after electroporation. (b) Normalized intracellular recorded amplitude for the first 60 s after electroporation. (c) Time plot of recorded action potentials by IrOx nanotubes show intracellular access for almost 1 h in a single recording session. Green arrows indicate sudden amplitude step drops. (d) Expanded views of the five amplitude drops. Red lines are drawn to guide eyes. (e) Statistical comparison of intracellular access duration between Au nanopillar and IrOx nanotube electrodes. IrOx nanotubes afford more than an order of magnitude longer intracellular access than Au nanopillars. (f) Distributions of drop durations. Figure 3b plots out the normalized amplitude of recorded action potentials by IrOx nanotubes (remains constant at 15.2±0.2 mV after 245 action potentials in 1 min) and by Au nanopillars (decays from 1.2 to 0.25 mV after 152 action potentials in 51 s). Surprisingly, IrOx nanotube electrodes have more than an order of magnitude longer intracellular access, sometimes achieving intracellular recording for almost an hour ( Fig. 3c ). We define the lifetime of intracellular access as the time when the amplitude decays to 20% of its initial amplitude. Statistical measurements over many cultures in Fig. 3d show that the IrOx nanotubes ( n =13) offer one-to-two orders of magnitude longer intracellular access duration than Au nanopillars ( n =19). Figure 3: Prolonged intracellular access duration by IrOx nanotube electrodes. ( a ) Intracellular recording of HL-1 action potentials by IrOx nanotube and Au nanopillar electrodes for the first 60 s after electroporation. ( b ) Normalized intracellular recorded amplitude for the first 60 s after electroporation. ( c ) Time plot of recorded action potentials by IrOx nanotubes show intracellular access for almost 1 h in a single recording session. Green arrows indicate sudden amplitude step drops. ( d ) Expanded views of the five amplitude drops. Red lines are drawn to guide eyes. ( e ) Statistical comparison of intracellular access duration between Au nanopillar and IrOx nanotube electrodes. IrOx nanotubes afford more than an order of magnitude longer intracellular access than Au nanopillars. ( f ) Distributions of drop durations. Full size image The improvements in intracellular access durations and the recorded signal amplitude allowed us to examine the membrane resealing in great detail. It is interesting to note that the decay of the measured action potential amplitudes is composed of both continuous decays and abrupt step drops. Figure 3c shows a stable recording of intracellular potentials for the first 30 min. In the next 25 min, the amplitude of the action potentials exhibited five sudden drops with 0.5, 1, 1.5 and 2 mV amplitudes ( Fig. 3e ). The amplitude of the action potential is relatively stable in between drops. Afterward, the amplitude decayed continuously and the recorded action potentials transited from intracellular shape to extracellular shape. As the recorded amplitude is linearly proportional to membrane pore conductance after electroporation ( Supplementary Note 2 and ref. 14 [14] ), the sudden drop in amplitude likely indicates the sudden sealing of membrane pores. Figure 3f quantifies the drop duration (time difference between two adjacent plateau endpoints) and reveals that half of the drops occurred in less than 2 s ( n =49). Cell membrane spontaneously protrudes into the nanotubes To understand the enhancement of recorded amplitude and the prolongation of intracellular access duration, we examined the cell–nanotube interface by scanning electron microscopy. For this purpose, we cultured HL-1 cardiomyocytes on a large array of IrOx nanotubes (see Methods section for the fabrication of large IrOx nanotube arrays). Scanning electron microscopy shows that cardiomyocytes engulf the vertical nanotube arrays. This tight interaction is most easily observed at the cell edges, where the cell thickness is smaller than the nanotube height ( Fig. 4a ). We observe that the top plasma membrane dips into the nanotube openings ( Fig. 4a arrow). To further study the interaction between the bottom membrane and the nanotubes at the cell centre, we removed the top membrane, the cell nucleus and cytosol by a brief sonication [35] , [36] . 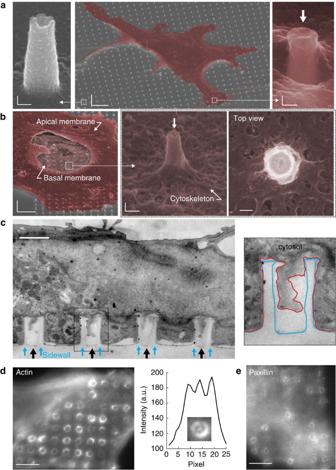Figure 4: Cardiomyocyte interfacing with the vertical nanotube arrays. (a) SEM images of a cardiomyocyte growing on top of a large IrOx nanotube array show that the cell engulfs the nanotubes. The top membrane dips into the nanotubes (white arrow) at the cell edge. Scale bars, left of panel 100 nm, centre of panel 5 μm, right of panel 100 nm. (b) SEM image of an unroofed cell with part of the top plasma membrane, the nucleus and the cytosol removed. Expanded images show the bottom membrane and cytoskeleton wrap around the IrOx nanotube and extends into the nanotube. Scale bars, left of panel 5 μm, centre of panel 200 nm, right of panel 100 nm. (c) TEM vertical section image of a cardiomyocyte growing on top of quartz nanotube arrays (black arrows) show that the bottom plasma membrane protrudes into the nanotubes. Inset shows the outline of a nanotube (blue line) and the plasma membrane (red line). Scale bar, 1 μm. (d) Immunofluorescent staining of F-actin reveals actin rings surrounding the outside of the quartz nanotubes. The expanded view and a line-plot across the centre of the nanotube clearly show the accumulation of the actin inside the nanotube. Scale bar, 4 μm. (e) Immunofluorescent staining of paxillin shows that some of the focal adhesions colocalize with the quartz nanotubes. Scale bar, 4 μm. Figure 4b and Supplementary Fig. 9 show that the bottom cytoskeleton wraps around the vertical nanotubes like a dented tent with the nanotubes as posts. The bottom membrane is seen to extend inside the vertical nanotubes. Figure 4: Cardiomyocyte interfacing with the vertical nanotube arrays. ( a ) SEM images of a cardiomyocyte growing on top of a large IrOx nanotube array show that the cell engulfs the nanotubes. The top membrane dips into the nanotubes (white arrow) at the cell edge. Scale bars, left of panel 100 nm, centre of panel 5 μm, right of panel 100 nm. ( b ) SEM image of an unroofed cell with part of the top plasma membrane, the nucleus and the cytosol removed. Expanded images show the bottom membrane and cytoskeleton wrap around the IrOx nanotube and extends into the nanotube. Scale bars, left of panel 5 μm, centre of panel 200 nm, right of panel 100 nm. ( c ) TEM vertical section image of a cardiomyocyte growing on top of quartz nanotube arrays (black arrows) show that the bottom plasma membrane protrudes into the nanotubes. Inset shows the outline of a nanotube (blue line) and the plasma membrane (red line). Scale bar, 1 μm. ( d ) Immunofluorescent staining of F-actin reveals actin rings surrounding the outside of the quartz nanotubes. The expanded view and a line-plot across the centre of the nanotube clearly show the accumulation of the actin inside the nanotube. Scale bar, 4 μm. ( e ) Immunofluorescent staining of paxillin shows that some of the focal adhesions colocalize with the quartz nanotubes. Scale bar, 4 μm. Full size image To further examine the nanotube–cell membrane interface, we conducted transmission electron microscopy (TEM) study on vertical sections. We employed large arrays of quartz nanotubes instead of IrOx nanotubes because IrOx is not compatible with the sample preparation for TEM that requires the dissolution of the nanotubes for resin embedding [17] . Previous studies by us have shown that different materials do not affect the cell–nanostructure interface because the surfaces are coated with fibronectin/gelatin [12] . The quartz nanotubes are slightly larger in diameter (~500 nm outer and ~400 nm inner diameter) than IrOx nanotubes to enhance the probability of obtaining vertical sections (80–100 nm thickness) through the centre of the nanotubes. Vertical sections cutting through the nanotubes clearly showed that the bottom plasma membrane protrudes into the nanotubes ( Fig. 4c ). The dark area indicates the cytosol. Statistics show that the gap between the cell membrane and the inner tube surface is generally larger than the gap between the cell membrane and the outer tube surface (analysis details of 15 nanotubes, 12 cells are shown in Supplementary Fig. 10 ). We performed immunofluorescence staining to examine the distribution of cellular proteins around nanotubes. Quartz nanotubes were used because the size of IrOx nanotubes is below the optical resolution. Staining of F-actin shows actin rings locked on the outside walls of the nanotubes. Enlarged images of a single nanotube also show actin inside the hollow centres of the quartz nanotubes ( Fig. 4d ). Staining of a focal adhesion protein paxillin shows that many focal adhesion points colocalized with the quartz nanotube arrays ( Fig. 4e ). All of the above observations suggest a tight cell–nanotube interaction at the molecular level. We hypothesize that the highly positive curvature of the membrane inside the nanotube is responsible for the prolonged intracellular access duration. To confirm this hypothesis, we compared the membrane pore sealing in a flat membrane versus that in a positively curved membrane ( Supplementary Fig. 11a,b ). A glass pipette electrode with ~450 nm inner diameter was gently pushed against the HL-1 cardiomyocyte membrane either without suction (flat membrane) or with suction to induce highly positively curved membrane inside the pipette. The seal resistances were kept at 25–30 MΩ in both configurations and gigaseals were deliberately avoided. Electric pulses were sent via the pipette to electroporate the patched membrane. Then, spontaneous action potential current was measured and its decays revealed the intracellular access duration ( Supplementary Fig. 11c ). Statistics show that positive membrane curvature gives a longer intracellular access duration ( n =15 in either configuration, P =0.0028). We note that this experiment mimics but does not exactly replicate our IrOx nanotube electrode recording, because it does not take into account the cytoskeleton reorganization on a longer timescale. Nevertheless, this experiment clearly demonstrates the significant effect of membrane curvature on intracellular access duration. Confirmation of nanotube intracellular recording We verified our IrOx nanotube electrode recording by simultaneous whole-cell current clamp recording on the same cells. We patched a cardiomyocyte that resided on top of the IrOx nanotubes ( Fig. 5a ) and exhibited spontaneous contraction ( Supplementary Movie 1 ). Before any electroporation, the patch clamp recorded a train of spontaneous action potentials with a −80 mV resting membrane potential and an amplitude of 100 mV (peak-to-baseline). At the same time, the IrOx nanotubes registered extracellular spikes about 300 μV peak-to-peak ( Fig. 5b ). After sending voltage pulses through the IrOx nanotubes, we observed sudden rising of the resting membrane potential by the patch-clamp recording ( Fig. 5c ), indicating cell membrane electroporation. After electroporation, the shape of the action potential was similar to that before the electroporation whereas the action potential duration at 50% depolarization was changed from 61 to 63 ms ( Supplementary Fig. 12 ). As time progressed for the next 5 min, the peak of the action potential measured by the whole-cell patch clamp remained almost constant while the resting membrane gradually repolarized and eventually returned to the pre-electroporation level, confirming membrane resealing. As expected, the recorded signal by IrOx nanotubes increased significantly and the action potential switched to intracellular shape ( Fig. 5c ), confirming membrane electroporation. Even though the amplitude of the action potentials recorded by IrOx nanotubes is much smaller than that recorded by patch clamp, they have almost identical waveforms throughout the recording ( Fig. 5d ). 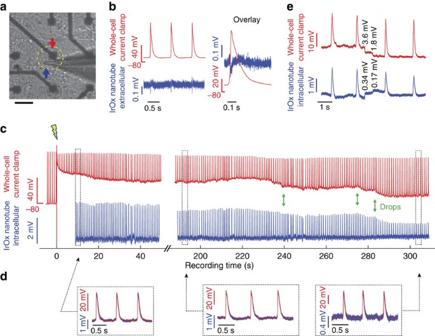Figure 5: Simultaneous recording by IrOx nanotube electrodes and patch clamp. (a) A bright field image of a cardiomyocyte (yellow dashed-line circle) being simultaneously recorded by the IrOx nanotubes (red arrow) and a patch pipette electrode (blue arrow). Scale bar, 20 μm. (b) Before electroporation, patch clamp records intracellular action potentials with −80 mV resting membrane potential, while IrOx nanotube records extracellular potentials that match the intracellular action potentials in the time domain but not in shape. (c) After local electroporation, IrOx nanotube records intracellular action potential. The time-dependent decay of the IrOx signal matches well with the decrease of the resting membrane potential recorded by patch clamp. (d) Intracellular recording by IrOx nanotubes matches well with intracellular recording by patch clamp after scaling. (e) Sudden drops in resting membrane potential detected by patch clamp are faithfully detected by IrOx nanotubes. Figure 5: Simultaneous recording by IrOx nanotube electrodes and patch clamp. ( a ) A bright field image of a cardiomyocyte (yellow dashed-line circle) being simultaneously recorded by the IrOx nanotubes (red arrow) and a patch pipette electrode (blue arrow). Scale bar, 20 μm. ( b ) Before electroporation, patch clamp records intracellular action potentials with −80 mV resting membrane potential, while IrOx nanotube records extracellular potentials that match the intracellular action potentials in the time domain but not in shape. ( c ) After local electroporation, IrOx nanotube records intracellular action potential. The time-dependent decay of the IrOx signal matches well with the decrease of the resting membrane potential recorded by patch clamp. ( d ) Intracellular recording by IrOx nanotubes matches well with intracellular recording by patch clamp after scaling. ( e ) Sudden drops in resting membrane potential detected by patch clamp are faithfully detected by IrOx nanotubes. Full size image The decay of the resting potentials recorded by patch clamp reflects membrane sealing, which also shows continuous decays and discontinuous drops. The sudden drops of the resting membrane potential in the whole-cell current clamp were faithfully detected as sudden amplitude drops by the IrOx nanotubes (green arrows in Fig. 5c ). The exact correspondence between the IrOx nanotube recording and the patch-clamp recording confirms that the membrane pores were highly localized around the nanotube electrodes. Figure 5e further illustrates that drops as fast as 20 ms can be faithfully recorded. Note that the amplifier for the IrOx recording has a high-pass filter of ~0.01 Hz and therefore did not register DC level of the action potentials (Multi Channel Systems). Nanometer-size pores are created by electroporation Finally, we estimated the size of the pores created by electroporation. Before nanotube electroporation, the HL-1 cardiomyocyte was held at −80 mV with −390 pA in a whole-cell current clamp, thus giving an input resistance of R m =205 MΩ for the intact cell membrane. As shown in Fig. 5c , the resting membrane potential depolarized to −35 mV 10 s after electroporation under the same whole-cell current clamp, which indicates that the input resistance dropped to 90 MΩ. Since this new input resistance is a parallel circuit of R m and R access + R seal ( Supplementary Fig. 13 and Supplementary Note 1 ), we calculated the R access + R seal to be 160 MΩ. To individually estimate the values of R access and R seal , we take into account that the amplitude of the action potential recorded by the nanotube electrode is V rec =3.5 mV at 10 s. From the circuit diagram, the V rec is related to V in as V rec = V in R seal /( R seal + R access ), where V in is the intracellular action potential recorded by whole-cell current clamp and V rec is the action potential recorded by nanotube electrode. From our data V in =30 mV and V rec =3.5 mV, we calculated R seal =19 MΩ for an array of nine nanotubes. The seal resistance for a single electrode is about 170 MΩ. The membrane access resistance is calculated to be R access =141 MΩ. Using the resistivity of physiological solution ρ =100 Ω cm and membrane thickness of l ~8 nm, we estimated the size of the hole using equation: r hole =( ρ l/ (π R access )) 1/2 and R access =141 MΩ at 10 s, the pore diameter is estimated to be 8.4 nm. To compute the pore size immediately after electropration, we used the membrane potential at this point of −15 mV to calculate R access + R seal =38 MΩ. We then obtained R access =19 MΩ and an equivalent pore diameter of 23 nm. We note that the diameter values are for either a single equivalent hole or a set of smaller pores. We also note that the previous work showed that the electroporation-induced pore size is in the range of ~25 nm immediately after electroporation [37] . In this study, we demonstrate that IrOx nanotube electrodes significantly improve both the sensitivity and the intracellular access duration compared with nanopillar electrodes. Compared with patch clamp, the advantages of nanotube electrodes for intracellular recording include easy scalability for simultaneous measurement of many cells, minimal invasiveness of the cell viability and longer-term monitoring of the same cell [9] , [11] . Unlike patch clamp, it does not require highly skilled manipulation or a microscope. Therefore the electrophysiology measurement is done while the cells are kept in a regular incubator. However, nanotube intracellular recording still suffers from lower signal amplitude and lower signal-to-noise ratio, and further development is needed to achieve comparable signal quality as patch clamp. The development of nanotube electrodes takes advantage of the cell’s intrinsic property to explore its surroundings. The contour of the cell membrane and the formation of focal adhesion are highly sensitive to geometrical and mechanical constraints from their extracellular microenvironment. For example, vertical nanopillars have been shown to curve membrane inward and stimulate cell adhesion, which results in a decreased membrane–electrode gap distance and a much higher seal resistance [16] , [17] . Protrusion of the cell membrane inside the nanotube electrode increases local membrane tension and is likely to further decrease the membrane–electrode gap distance. Furthermore, the flux of ions from those ion channels or pores that are on the membrane inside the nanotubes is more likely to be detected by the electrode before leaking to the bulk medium. We attribute the drastic increase of intracellular access duration for nanotube electrode to the highly positive curvature of the membrane inside the nanotube. Sealing of the membrane pores could be significantly affected by the membrane curvature in two ways. First, the line tension surrounding the lipid membrane pore is the driving force for the closure of the pore in the absence of proteins [38] . Previous studies show that membrane tension such as high positive membrane curvature stimulates pore formation and decreases the line tension force for pore closure [39] , [40] . Second, in a live cell, the membrane repair involves fusion of intracellular vesicles with the plasma membrane [41] , [42] . Membrane curvature plays an important role in lipid and protein sorting [43] . For example, negative membrane curvature induced by nanocones has shown to recruit many BAR-domain containing proteins and stimulates endocytosis events [36] . Curvature-induced distinct protein and lipid compositions on positive curvature (membrane inside the nanotube) and on negative curvature (membrane wrapping around nanopillars or the outside of nanotubes) could possibly account for the significantly increased intracellular access duration by IrOx nanotube electrodes. Pt contact pad fabrication A four-inch quartz wafer was diced into 20 × 20 mm 2 pieces, and each piece was patterned with eight-by-eight arrays of 8 × 8 μm 2 electrode pads and 3 μm wide lead lines using photolithography, 80 nm/10 nm Pt/Ti deposition and liftoff. The substrate surface was subsequently covered with a 250 nm Si 3 N 4 and 50 nm SiO 2 layer by plasma-enhanced chemical vapour deposition (STS). The Pt contact pads on the edge of the chip were exposed by plasma etching the covering Si 3 N 4 /SiO 2 with CHF 3 /O 2 chemistry (Drytek). The parasitic capacitance of the Pt line in phosphate-buffered saline was measured to be 3.8 pF and the current leakage during electrophysiology measurement was minimal. Subsequently, three-by-three arrays of nanoholes were defined by electron beam lithography (Raith150) at 20 kV on a 700-nm thick ZEP520 resist (Zeon) spun on the chip. The Si 3 N 4 /SiO 2 beneath the nanoholes was removed by CHF 3 /O 2 plasma etching (Drytek) until the underlying Pt was exposed. IrOx nanotubes were subsequently electrodeposited with the Si 3 N 4 /SiO 2 layer and the remaining resist as the template. Iridium oxide nanotube electrodeposition Electroplating bath consisted of 74 mg iridium(IV) chloride hydrate and 202 mg oxalic acid dihydrate in 50 ml Millipore water. The pH was then raised to 10.5 by adding 700 mg potassium carbonate [23] , [26] (Sigma-Aldrich). The solution was allowed to equilibrate at room temperature for at least 48 h. During this process, the solution colour turned from dark green to dark purple. IrOx was then anodically electrodeposited into the nanoholes as well as the Pt contact pads with 0.1 mA DC current and a 5 cm 2 Pt sheet as the counter electrode. Because the total contact pad area (~50 mm 2 ) was much larger than the total nanohole area (~34 μm 2 ), the electrodeposition was very consistent among chips. Finally, the ZEP520 resist was removed by Remover PG (Microchem) and the chip was interfaced to a custom designed printed circuit board [12] . For characterization studies, IrOx nanotubes were also electroplated on glass coverslips coated with Au/Cr (20 nm/5 nm) patterned with large arrays of ZEP520 resist nanoholes. Au nanopillars were electrodeposited with 0.1 mA DC current in 24 K pure gold solution (Gold Plating Services). The nanopillars have the same height as the IrOx nanotubes and the nanopillars diameters were adjusted such that the nanopillars and nanotubes have the same surface area. Nanotube characterization Scanning electron microscopy images were taken by dual-beam FIB/SEM system (Strata 235DB, FEI) and false coloured by GIMP. For surface element identification, nanotubes electrodeposited on Au/Cr covered glass coverslip were examined by Auger electron spectroscopy (Phi 700, ULVAC-PHI) at 20 kV. Post acquisition analysis included 9-point Savitzky–Golay smooth and derivative. Electrochemical impedance spectroscopy and cyclic voltammetry of nanoelectrodes in phosphate-buffered saline were performed by Agilent 4294A precision impedance analyser and Agilent B1500A analyser (Agilent Technologies), respectively. Nanotube geometry measurement We defined 50 × 50 nanohole arrays, each in a 100 × 100 μm 2 area, by electron beam lithography on ZEP520 resist on coverslips without any underlying Pt connections. IrOx nanotubes electrodeposited in this nanohole template are uniform in both size and shape ( Supplementary Fig. 2a ). We randomly picked thirty nanotubes to measure their diameters and wall thickness by SEM line scans ( Supplementary Fig. 2b ). Nanotube diameter is defined as the separation between the two intensity peaks; and wall thickness is defined as the full width at half maximum at each peak. The average nanotube radius is 90.7±1.4 nm and the average wall thickness is 39.8±3.0 nm ( n =30) for an electron beam lithography write radius of 70 nm and exposure dose of 250 μC cm −2 at 20 kV. By writing other diameters, we can fabricate IrOx nanotubes of different diameters. HL-1 and primary rat cardiomyocyte culture Each device was cleaned by 10 min oxygen plasma (Drytek) and coated with 10 μg ml −1 fibronectin in 0.02% w/w gelatin solution overnight. HL-1 cells were then plated inside the chamber at a density of 10 4 cm −2 and maintained in the Claycomb medium supplemented with 10% fetal bovine serum, 0.1 mM norepinephrine, 2 mM L -glutamine and 100 U ml −1 penicillin and 100 mg ml −1 streptomycin in a 37 °C incubator with 5% CO 2 . Medium was changed daily. Cell viability test was performed with 1 μM calcein AM and 1 μM propidium iodide after washing the cells three times with phosphate-buffered saline. For primary culture, 18-day-pregnant female rats were anaesthetized and then euthanized by a combination of excess CO 2 and cervical dislocation. Embryos were removed and collected in HBSS. Subsequently, embryonic hearts were extracted, minced and dissociated in 0.25% trypsin at 37 °C for 30 min. The tissues were triturated and plated on the nanotube devices. These protocols agree with Stanford Administrative Panel on Laboratory Animal Care. Cells were maintained with DMEM (Dulbecco’s Modified Eagle Medium) solution supplemented with 10% fetal bovine serum, 2 mM L -glutamine, and 100 U ml −1 penicillin and 100 mg ml −1 streptomycin in a 37 °C incubator with 5% CO 2 . All experimental data were collected on HL-1 cardiomyocytes except Supplementary Fig. S7 . Immunostaining and electron microscopy HL-1 cardiomyocytes cultured on quartz nanotubes were fixed in 4% paraformaldehyde in PBS at room temperature for 15 min, permeabilized in 1% Triton X-100 in PBS for 5 min, and blocked in 0.3% Triton X-100 and 1% BSA in PBS for 1 h. The specimen was then incubated with mouse anti-paxillin antibody (BD Bioscience) in 1:500 dilution for 1 h and subsequently incubated with ActinGreen 488 (Life Technology) and anti-mouse antibody for 1 h and finally imaged by an inverted microscope (Leica DMI6000 B). For SEM study, the HL-1 cells cultured on the IrOx nanotubes were fixed with 2% glutaraldehyde and 4% paraformaldehyde in 0.1 M sodium cacodylate buffer (pH 7.4) and post-fixed in 1% osmium tetroxide in the same buffer at 4 °C for 1 h. Chemicals were from Electron Microscopy Sciences. After rinsing, the sample was dehydrated in a graded ethanol series (50, 70, 80, 95 and 100%) and dried in a liquid CO 2 critical point dryer (Autosamdri 815b, Tousimis). The sample was then sputter-coated with a 4 nm Cr layer to improve conductance and imaged by electron microscope (Raith150, Raith and Strata 235DB, FEI). In the unroofing experiment, the HL-1 cells cultured on the IrOx nanotubes were fixed for 20 min and transferred to a beaker with phosphate-buffered saline. The sample was then ultrasonicated by a probe positioned ~7 mm above the surface for 2–3 s with 20% amplitude [35] (Sonic Dismembrator FB-505, Fisher Scientific). The sample was then transferred back to the fixative and underwent rest of the electron microscopy preparation. For TEM study, the HL-1 cells cultured on the quartz nanotubes were fixed in the same buffer, stained first with 1% OsO 4 and 0.8% potassium ferricyanide in 0.1 M sodium cacodylate on ice for 2 h and then with 1% uranyl acetate at 4 °C overnight. The sample was dehydrated in the graded ethanol series and embedded in Epon. The quartz was dissolved in hydrofluoric acid and reembedded on the bottom side. The sample was then sectioned into <100 nm sections and finally imaged at 120 kV on TEM (JEOL JEM-1400). Quartz nanotube fabrication Arrays of 100-nm thick Cr nanorings were patterned on quartz coverslips by electron beam lithography, metal deposition and liftoff. Using these nanorings as masks, quartz nanotubes were created by reactive ion etch with CHF 3 and O 2 chemistry (AMT 8100 etcher, Applied Materials). The residual Cr was removed by CR-14 etchant. Electrophysiology recording After the HL-1 cells exhibited spontaneous beating (usually four days after plating), the chip was connected to a 60-channel voltage amplifier (MEA1060-Inv, Multi Channel Systems) for recordings at 5 kHz sampling rate. The recordings were performed in Claycomb culture medium at room temperature. The electroporation pulse consisted of 100 consecutive biphasic and symmetric square pulses, each with 400 μs period and 3.5 V amplitude. Recordings were resumed ~10 s after electroporation to avoid amplifier saturation. Nanotube electrode devices were reused after multiple cultures by trypsinization, deionized water clean and oxygen plasma. Whole-cell current clamp was performed at room temperature using Axon Multiclamp 700B amplifier (Molecular Devices). Patch pipettes had resistance of 2–4 MΩ. Intracellular solution contained (in mM): 140 KCl, 10 NaCl, 10 HEPEs and 1 EGTA (pH 7.3) and extracellular batch solution was Claycomb medium. Data were sampled at 10 kHz and low-pass filtered at 3 kHz by Axon Digidata 1440A (Molecular Devices). For electrophysiology recording of membrane sealing on flat membrane versus positively curved membrane, we fabricated glass pipettes with ~450 nm inner diameter and access resistance of 9–11 MΩ when filled with intracellular solution. For the flat membrane configuration, the pipettes were gently pushed against the HL-1 cardiomyocyte membrane without suction. For the positively curved membrane configuration, gentle suction was applied through the pipette. Seal resistances were in the range of 25–30 MΩ in both configurations. Five electroporation pulses were applied through the pipette electrode to electroporate the patched membrane. In voltage clamp mode, square waves with 10 mV amplitude of 1 kHz frequency were applied and the resultant current passing through the pipettes was monitored. The spontaneous action potential current was detected as spikes in the recorded current. How to cite this article: Lin, Z. C. et al. Iridium oxide nanotube electrodes for highly sensitive and prolonged intracellular measurement of action potentials. Nat. Commun. 5:3206 doi: 10.1038/ncomms4206 (2014).